Gold-in-copper at low *CO coverage enables efficient electromethanation of CO2 The renewable-electricity-powered CO 2 electroreduction reaction provides a promising means to store intermittent renewable energy in the form of valuable chemicals and dispatchable fuels. Renewable methane produced using CO 2 electroreduction attracts interest due to the established global distribution network; however, present-day efficiencies and activities remain below those required for practical application. Here we exploit the fact that the suppression of *CO dimerization and hydrogen evolution promotes methane selectivity: we reason that the introduction of Au in Cu favors *CO protonation vs. C−C coupling under low *CO coverage and weakens the *H adsorption energy of the surface, leading to a reduction in hydrogen evolution. We construct experimentally a suite of Au-Cu catalysts and control *CO availability by regulating CO 2 concentration and reaction rate. This strategy leads to a 1.6× improvement in the methane:H 2 selectivity ratio compared to the best prior reports operating above 100 mA cm −2 . We as a result achieve a CO 2 -to-methane Faradaic efficiency (FE) of (56 ± 2)% at a production rate of (112 ± 4) mA cm −2 . The CO 2 electroreduction reaction (CO 2 RR) to valuable fuels and feedstocks, powered using renewable electricity, offers a sustainable approach to store intermittent renewable energy [1] . Prior CO 2 RR studies have reported the generation of C 1 to C 3 chemicals such as CO, methane, formate, ethylene, ethanol, and n-propanol [2] , [3] , [4] , [5] , [6] , [7] , [8] , [9] , [10] . Among these products, carbon-neutral methane produced from CO 2 RR is desired due to well-established natural gas infrastructure [11] . Practical CO 2 RR systems need to produce a desired product with high selectivity, conversion rate, and energy efficiency (EE) [12] , [13] . In prior reports, most advances in improving the selectivity to methane in CO 2 RR operate at current densities below 50 mA cm −2 (ref. [14] , [15] , [16] , [17] , [18] ). Techno-economic analyses suggest that compelling CO 2 RR systems require current densities above 100 mA cm −2 (ref. [19] ), which prompted us to concentrate on improving the performance of CO 2 RR to methane in high current density regimes (>100 mA cm −2 ). In CO 2 RR, *CO protonation to *CHO is the potential-determining step for methane formation, and it competes with C–C coupling toward C 2 products [20] , [21] . In addition, *CO protonation competes with the hydrogen evolution reaction (HER), since both need *H (ref. [22] ). The simultaneous suppression of both HER and C–C coupling will improve methane selectivity. Early studies by Hori et al. [2] showed that Cu is the transition metal catalyst that generates methane and C 2+ products; but that it did so with low product selectivity. Introducing a second metal into Cu has been shown to be a promising route to tune the product selectivity in CO 2 RR (refs. [23] , [24] , [25] , [26] , [27] , [28] , [29] , [30] ). Prior studies report that Au–Cu bimetallic catalysts of varying structures exhibit good selectivity to CO or alcohols, albeit with pure CO 2 feeds (refs. [31] , [32] , [33] , [34] ). Here we present a strategy wherein we regulate *CO availability on Au–Cu catalysts, enabling selectivity to methane at high production rates in CO 2 RR. Density functional theory (DFT) calculations indicate that the introduction of Au in Cu not only steers the selectivity from C–C coupling to *CO protonation under low *CO coverage, but also tends to suppress HER relative to Cu. By implementing this concept experimentally, we achieve an FE of (56 ± 2)% to methane. 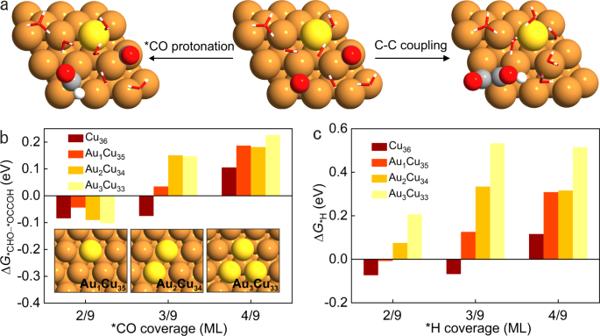Fig. 1: DFT studies. aGeometries of *CO, *CHO, and *OCCOH intermediates on Au–Cu surface, showing the competitive steps of *CO protonation and C–C coupling.bReaction free energy difference between *CO protonation and C–C coupling steps on Cu36, Au1Cu35, Au2Cu34, and Au3Cu33surfaces under varying *CO coverages.cReaction free energies for *H intermediate formation under varying *H coverages on Cu36, Au1Cu35, Au2Cu34, and Au3Cu33surfaces. Cu, Au, C, O, and H atoms in Fig.1are illustrated as orange, yellow, grey, red, and white spheres, respectively, while the water molecules are shown as sticks. Source data are provided as a Source Data file. The methane:H 2 selectivity ratio is improved 1.6× compared with prior reports having a total current density above 100 mA cm −2 (Supplementary Table 1 ) (refs. [35] , [36] , [37] , [38] , [39] ). DFT calculations In a previous study, we found that lowering the *CO coverage on a Cu surface improved the selectivity to methane in CO 2 RR while still suffering from prominent HER (ref. [35] ). Introducing a second element to Cu, such as Ag, has been shown to suppress HER (refs. [21] , [28] ). Au—like Ag—has a greater free energy of hydrogen adsorption than Cu, suggesting that it is also a poor HER catalyst [40] . We thus use Au–Cu as a representative example to assess methane selectivity on catalysts with HER-suppressing dopants under different *CO coverages. In addition, we note that selecting an element that is on the same side of the hydrogen adsorption volcano curve as Cu avoids any synergistic effects that may optimize the *H binding energy leading to better HER, such as with Cu–Ni or Cu–Pt (refs. [41] , [42] , [43] ). Computationally, we built three Au–Cu surfaces by replacing one, two, or three surface Cu atoms of a (3 × 3 × 4) Cu(111) supercell with Au atoms, denoted Au 1 Cu 35 , Au 2 Cu 34 , and Au 3 Cu 33 , respectively. With DFT, we first calculated the reaction free energies of *CO to *CHO (∆ G *CHO ) for methane formation and C–C coupling (∆ G *OCCOH ) for C 2 products on these Au–Cu surfaces under different *CO coverages (Fig. 1a , Supplementary Figs. 1 – 4 , and Supplementary Tables 2 and 3 ). ∆ G *CHO –∆ G *OCCOH is used as a descriptor of the propensity for *CO protonation vs. C–C coupling. We found that the values of ∆ G *CHO –∆ G *OCCOH on Au–Cu surfaces decrease when one reduces *CO coverage from 4/9 to 2/9 monolayer (ML) (Fig. 1b ), a trend similar to that on Cu. Thus lowering *CO coverage on Au–Cu surfaces is predicted to favor methane vs. C 2 products, as previously shown on Cu (ref. [35] ). In addition, DFT calculation results show that the values of ∆ G *CHO –∆ G *OCCOH on Au–Cu surfaces are not always lower than the values of ∆ G *CHO –∆ G *OCCOH on Cu at different *CO coverages (Fig. 1b ), suggesting that only under low *CO coverage do some Au–Cu surfaces show a higher ratio of methane to C 2 products compared to Cu. Fig. 1: DFT studies. a Geometries of *CO, *CHO, and *OCCOH intermediates on Au–Cu surface, showing the competitive steps of *CO protonation and C–C coupling. b Reaction free energy difference between *CO protonation and C–C coupling steps on Cu 36 , Au 1 Cu 35 , Au 2 Cu 34 , and Au 3 Cu 33 surfaces under varying *CO coverages. c Reaction free energies for *H intermediate formation under varying *H coverages on Cu 36 , Au 1 Cu 35 , Au 2 Cu 34 , and Au 3 Cu 33 surfaces. Cu, Au, C, O, and H atoms in Fig. 1 are illustrated as orange, yellow, grey, red, and white spheres, respectively, while the water molecules are shown as sticks. Source data are provided as a Source Data file. Full size image To compare the HER activities on Cu and Au–Cu surfaces, we calculated the reaction free energies of *H intermediate formation (∆ G *H ) (Fig. 1c and Supplementary Fig. 5 ). The results suggest that Au–Cu surfaces tend to suppress HER compared to Cu under high *H coverages (Fig. 1c ). Taken together, these DFT studies suggest that Au–Cu tends to promote methane selectivity with low *CO coverage, since this will suppress C–C coupling; and that Au–Cu will further advance CO 2 RR over HER compared to pure Cu. Preparation and characterization of catalysts To achieve the goal of high selectivity to methane in CO 2 RR with high current densities, we sought to fabricate Au–Cu catalysts. We used a galvanic replacement approach enabled by the differing reduction potentials of Au and Cu (ref. [44] ). Firstly, we prepared a 100 nm thick layer of Cu catalysts on the surface of polytetrafluoroethylene (PTFE) nanofibers via sputter deposition (Supplementary Figs. 6 and 7 ). We then immersed the Cu/PTFE in an N 2 -saturated HAuCl 4 aqueous solution at 65 °C for 15 min to prepare the Au–Cu catalysts on PTFE as the electrodes (Fig. 2a–d ) via the galvanic replacement between Cu and AuCl 4 − —this approach allows us to directly tune the ratio of Au and Cu on PTFE substrates. Fig. 2: Structural and compositional analyses of 7% Au–Cu catalysts on PTFE. a Low magnification secondary electron image (above) and the corresponding backscattered electron image (below) of the 7% Au–Cu/PTFE, showing the dispersed Au nanoparticles (bright spots). b Secondary electron image and the corresponding EDX elemental mapping of Au and Cu for the 7% Au–Cu/PTFE. c High-angle annular dark-field scanning transmission electron microscopy (HAADF-STEM) image of one 7% Au–Cu/PTFE nanofiber. d High-magnification bright-field STEM image and the corresponding elemental mapping of Au and Cu from a section of one 7% Au–Cu/PTFE nanofiber. e , f High-resolution XPS spectra of Cu 2 p ( e ) and Au 4 f ( f ) for 7% Au–Cu/PTFE. Full size image Low-magnification scanning electron microscope (SEM) images and energy-dispersive X-ray spectroscopy (EDX) elemental mapping show a uniform distribution of elemental Cu and Au on PTFE nanofibers, accompanied by loosely distributed Au nanoparticles also on the nanofibers (Fig. 2a, b ). The bright-field scanning transmission electron microscope (STEM) image with higher magnification and corresponding EDX elemental mapping further confirms that Au and Cu are distributed evenly on the PTFE nanofibers (Fig. 2d ). High-resolution X-ray photoelectron spectroscopy (XPS) characterization of Au–Cu electrodes shows the presence of Au 0 and Cu which has been partially oxidized to Cu + in the air (Fig. 2e, f and Supplementary Figs. 8 and 9 ) [45] . The atomic percentage of Au in the catalyst surface is approximately 7% determined by XPS (denoted 7% Au–Cu), which is lower than previously reported Au–Cu alloy catalysts studied in CO 2 RR (refs. [31] , [32] , [33] ). Investigation of CO 2 electroreduction The CO 2 RR experiments were performed in a flow cell reactor with a three-electrode configuration (Supplementary Figs. 10 and 11 ) using CO 2 -saturated 1 M KHCO 3 aqueous solution as the electrolyte. Previous studies show that, in CO 2 RR, both reaction rate—determined by current density—and CO 2 concentration affect the concentration of *CO on the catalyst surface [35] . We thus evaluated the CO 2 RR performance of 7% Au–Cu electrodes by supplying gas streams consisting of different volume ratios of CO 2 to N 2 (Fig. 3 , Supplementary Figs. 12 and 13 , and Supplementary Table 4 ). Fig. 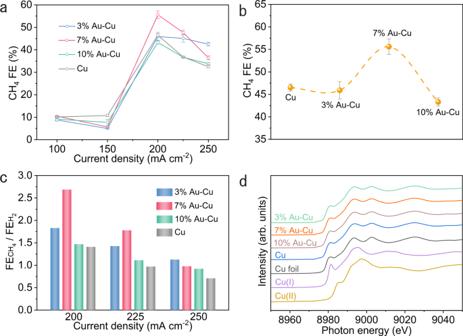Fig. 4: CO2RR performance at 84% CO2and operando XAS characterization. aMethane FEs on different catalysts at 84% CO2.bComparison of methane FEs on different catalysts at 200 mA cm−2. Error bars represent the standard deviation based on three separate measurements.cComparison of\({\rm{FE}}_{{\rm{CH}}_{4}}/{\rm{FE}}_{{\rm{H}}_{2+}}\)ratios on different catalysts at 84% CO2.dOperando Cu K-edge XANES spectra of different catalysts during CO2RR with a constant current density of 200 mA cm−2. Bulk Cu foil, Cu2O, and CuO are listed as references. 3: CO 2 RR performance of 7% Au–Cu catalysts at various CO 2 concentrations. a Methane FEs on 7% Au–Cu at various CO 2 concentrations. b Ethylene FEs on 7% Au–Cu at various CO 2 concentrations. c CH 4 cathodic EEs at different current densities under different CO 2 concentrations. d Comparison of \({\rm{FE}}_{{\rm{CH}}_{4}}/{\rm{FE}}_{{\rm{C}}_{2+}}\) ratios on 7% Au–Cu catalysts at various CO 2 concentrations. Error bars represent the standard deviation based on three separate measurements. 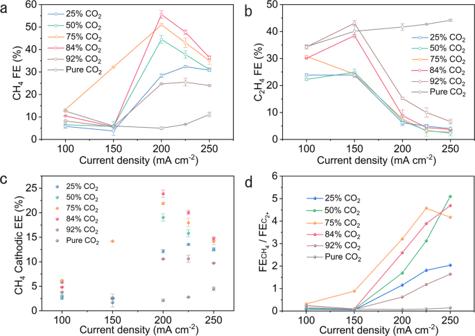Full size image Figure 3a, b shows FEs of methane and ethylene on 7% Au–Cu catalysts in the current density range of 100–250 mA cm −2 at various CO 2 concentrations (25% CO 2 , 50% CO 2 , 75% CO 2 , 84% CO 2 , 92% CO 2 , and pure CO 2 ). Fig. 3: CO2RR performance of 7% Au–Cu catalysts at various CO2concentrations. aMethane FEs on 7% Au–Cu at various CO2concentrations.bEthylene FEs on 7% Au–Cu at various CO2concentrations.cCH4cathodic EEs at different current densities under different CO2concentrations.dComparison of\({\rm{FE}}_{{\rm{CH}}_{4}}/{\rm{FE}}_{{\rm{C}}_{2+}}\)ratios on 7% Au–Cu catalysts at various CO2concentrations. Error bars represent the standard deviation based on three separate measurements. At low current densities (≤150 mA cm −2 ), 7% Au–Cu delivers appreciable ethylene FEs under pure CO 2 and CO 2 –N 2 mixed streams (Fig. 3b ). However, at high current densities (200–250 mA cm −2 ), relative to pure CO 2 , the methane FEs on 7% Au–Cu catalysts increase sharply in CO 2 –N 2 mixed streams while the ethylene FEs decrease dramatically, which we ascribe to the low *CO coverage on catalyst surfaces as a result of the reduced CO 2 concentration and high reaction rate. We note that, once they reach their peaks in these mixed streams, the methane FEs start to decrease with further increase in current density (Fig. 3a ), a finding we attribute to the lack of *CO for the *CO protonation step of methane formation [46] . In particular, at 84% CO 2 , we achieve the highest CH 4 FE of (56 ± 2)% on 7% Au–Cu catalysts with a CH 4 production rate of (112 ± 4) mA cm −2 . We calculated the CH 4 cathodic EEs at different current densities under different CO 2 concentrations (Fig. 3c ): the highest CH 4 cathodic EE of (24 ± 1)% was achieved at 200 mA cm −2 under 84% CO 2 . To evaluate experimentally the selectivity between *CO protonation and C−C coupling reaction steps, we further calculated the ratios of methane FE to total C 2+ FE ( \({{\rm{FE}}}_{{{{\rm{CH}}}}_{4}}/{{\rm{FE}}}_{{\rm{C}}_{2+}}\) ) on 7% Au–Cu catalysts at various CO 2 concentrations (Fig. 3d ). With low reaction rates (≤150 mA cm −2 ), the C 2+ selectivity is higher than the methane selectivity regardless of the CO 2 concentration. Under high current densities (200–250 mA cm −2 ), the \({\rm{FE}}_{{\rm{CH}}_{4}}/{\rm{FE}}_{{\rm{C}}_{2+}}\) ratio on 7% Au–Cu catalysts in CO 2 –N 2 mixed streams is much greater than that in pure CO 2 , suggesting that low *CO coverage on the surface of Au–Cu catalysts—as a consequence of a reduced CO 2 concentration and high current density—promotes the *CO protonation step for methane production, consistent with our DFT calculations. To explore the effect of Au concentration on CO 2 RR performance under CO 2 –N 2 co-feeds, we also prepared 3% Au–Cu and 10% Au–Cu catalysts on PTFE through a similar galvanic replacement approach (Supplementary Figs. 7 and 14 – 19 ) and measured CO 2 RR performance of the 3% Au–Cu, 10% Au–Cu, and Cu catalysts at 84% CO 2 for comparison (Fig. 4a–c , Supplementary Figs. 20 and 21 , and Supplementary Table 5 ). At low reaction rates (≤150 mA cm −2 ), the methane FEs on 3% Au–Cu, 7% Au–Cu, 10% Au–Cu, and Cu catalysts are below 11% (Fig. 4a ), while ethylene and ethanol are the main CO 2 RR products on these catalysts (Supplementary Fig. 20c and Supplementary Table 5 ). At high reaction rates (200–250 mA cm −2 ), methane becomes the main CO 2 RR product while ethylene FEs are below 12% on the 3% Au–Cu, 10% Au–Cu, and Cu catalysts; methane FEs on 3% Au–Cu, 10% Au–Cu, and Cu catalysts give peak values at 200 mA cm −2 and then decrease along with the increase in current density (Fig. 4a ). These trends are similar to that observed on the 7% Au–Cu catalysts. By comparing the highest methane FEs on different catalysts, we note that, among the catalysts studied, only 7% Au–Cu catalysts deliver higher methane FE vs. Cu catalysts (Fig. 4b ), suggesting the significance of controlling Au concentration in Au–Cu catalysts for promoting methane selectivity. The 7% Au–Cu delivers—compared to 3% Au–Cu and 10% Au–Cu—higher methane FE at 200 mA cm −2 . We associate this with improved suppression of HER on 7% Au–Cu (Supplementary Fig. 20a ) and note that both HER and *CO coverage impact methane FE. We also calculated the \({\rm{FE}}_{{\rm{CH}}_{4}}/{\rm{FE}}_{{\rm{C}}_{2+}}\) ratios on Cu and three Au–Cu catalysts at 84% CO 2 : only at high current density—low *CO coverage—do some of Au–Cu catalysts show higher \({{\rm{FE}}}_{{{{\rm{CH}}}}_{4}}/{{\rm{FE}}}_{{\rm{C}}_{2+}}\) ratios compared to Cu, in agreement with DFT calculations. Fig. 4: CO 2 RR performance at 84% CO 2 and operando XAS characterization. a Methane FEs on different catalysts at 84% CO 2 . b Comparison of methane FEs on different catalysts at 200 mA cm −2 . Error bars represent the standard deviation based on three separate measurements. c Comparison of \({\rm{FE}}_{{\rm{CH}}_{4}}/{\rm{FE}}_{{\rm{H}}_{2+}}\) ratios on different catalysts at 84% CO 2 . d Operando Cu K-edge XANES spectra of different catalysts during CO 2 RR with a constant current density of 200 mA cm −2 . Bulk Cu foil, Cu 2 O, and CuO are listed as references. Full size image At high current densities (200–250 mA cm −2 ) with high methane selectivity, the H 2 FEs on 3% Au–Cu, 7% Au–Cu, and 10% Au–Cu catalysts are lower than that on the Cu catalysts (Supplementary Fig. 20a ), suggesting that the introduction of Au in Cu tends to suppress HER when using dilute CO 2 feeds. We further calculated the ratio of methane FE to H 2 FE ( \({\rm{FE}}_{{\rm{CH}}_{4}}/{\rm{FE}}_{{\rm{H}}_{2}}\) ) on catalysts in high current density regimes (Fig. 4c ): compared with Cu catalysts, 3% Au–Cu, 7% Au–Cu, and 10% Au–Cu catalysts exhibit higher \({\rm{FE}}_{{\rm{CH}}_{4}}/{\rm{FE}}_{{\rm{H}}_{2}}\) ratios—with the highest value of 2.7 on 7% Au–Cu catalysts— indicating that the Au–Cu catalysts shifted the reaction from undesired HER toward *CO protonation for methane production. To investigate the chemical state of Cu in the catalysts during CO 2 RR, we carried out operando X-ray absorption spectroscopy (XAS) at the Cu K-edge at a constant current density of 200 mA cm −2 with an 84% CO 2 feed (Fig. 4d ). The average valence states of Cu in 3% Au–Cu, 7% Au–Cu, 10% Au–Cu, and Cu catalysts are zero during CO 2 RR, demonstrating that the difference in product selectivity among these catalysts is associated with the metallic state of Cu in lieu of copper oxides [5] , [47] . This work demonstrates that the introduction of Au in Cu facilitates *CO protonation for methane formation using CO 2 –N 2 co-feeds and suppresses HER at high current densities. DFT results show that a decrease in *CO coverage on Au–Cu surfaces favors *CO protonation vs. C–C coupling; compared with Cu, Au–Cu suppresses HER, enabling methane selectivity improvements under dilute CO 2 streams. Experimentally, we fabricated Au–Cu catalysts and regulated *CO availability by controlling the CO 2 concentration and current density, wherein the selectivity ratio of methane to H 2 exhibited the highest value of 2.7. We report a CO 2 -to-methane conversion with a high methane FE of (56 ± 2)% at a partial current density of (112 ± 4) mA cm −2 with a CO 2 –N 2 co-feed. These findings suggest a promising strategy to convert CO 2 to carbon-neutral methane with a combination of high selectivity, high conversion rate, and high cathodic EE through catalyst design and tuning local *CO coverage. DFT calculations In the Vienna ab initio simulation package, the generalized gradient approximation and the Perdew–Burke–Ernzerhof exchange-correlation functional was implemented for all DFT calculations [48] , [49] , [50] , [51] , [52] . The projector-augmented wave (PAW) method was used to treat the electron–ion interactions [53] , [54] with an energy cut-off of 450 eV for the plane-wave basis set. The force and energy convergence for all DFT calculations were set to 0.01 eV Å −1 and 10 −5 eV, respectively. A (3 × 3 × 4) Cu(111) supercell with the bottom two layers fixed was used to simulate the exposed Cu surface with a 15 Å vacuum gap. One, two, or three surface Cu atoms were substituted by Au atoms in the Au 1 Cu 35 , Au 2 Cu 34 , and Au 3 Cu 33 , respectively. A (3 × 3 × 1) Monkhorst–Pack k -points grid was used to optimize all the surface structures. In DFT calculations, we did not consider the isolated arrangement of Au dopants in Cu as the XAS characterization of the Au–Cu catalysts showed that Au atoms were not atomically dispersed in Cu (Supplementary Fig. 22 and Supplementary Table 6 ). Surface *CO coverages of 2/9 ML, 3/9 ML, and 4/9 ML were studied, where 2/9 ML corresponds to two single-carbon adsorbed species or one double-carbon species on the surface of the supercell. To systematically determine the most stable geometry of each reaction intermediate in CO 2 RR and HER under different *CO coverages (2/9, 3/9, and 4/9 ML) on different surfaces (Cu 36 , Au 1 Cu 35 , Au 2 Cu 34 , and Au 3 Cu 33 ), we considered different possibilities of *CO adsorption, protonation, and C–C coupling, as well as different directions of *OCCO protonation (more details of our computational workflow in Supplementary Fig. 23 ). We note that the models reported in this study include a charged water layer, i.e., an ML of six water molecules, one of which is a hydronium or charged water (H 3 O + ) molecule, to consider both field and solvation effects [55] . 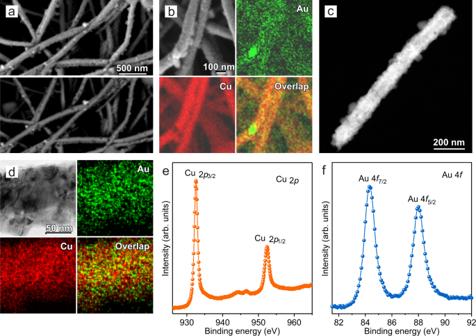The water structure was determined by ab initio molecular dynamics and adopted from a previous study [56] . The two competing CO 2 RR reaction steps as listed below [57] , [58] , [59] , [60] , [61] were simulated for the three *CO coverages while *H adsorption was simulated for equivalent *H coverages 
    ∗CO+H_2O+e^-→∗CHO+OH^-
 (1) 
    ∗CO+∗CO+H_2O+e^-→∗OCCOH+OH^-
 (2) 
    H^++e^-+∗→∗H
 (3) The Gibbs free energy changes (∆ G ) for *CO protonation, C–C coupling, and *H adsorption were calculated without dipole corrections based on the computational hydrogen electrode (CHE) model [62] . Fig. 2: Structural and compositional analyses of 7% Au–Cu catalysts on PTFE. aLow magnification secondary electron image (above) and the corresponding backscattered electron image (below) of the 7% Au–Cu/PTFE, showing the dispersed Au nanoparticles (bright spots).bSecondary electron image and the corresponding EDX elemental mapping of Au and Cu for the 7% Au–Cu/PTFE.cHigh-angle annular dark-field scanning transmission electron microscopy (HAADF-STEM) image of one 7% Au–Cu/PTFE nanofiber.dHigh-magnification bright-field STEM image and the corresponding elemental mapping of Au and Cu from a section of one 7% Au–Cu/PTFE nanofiber.e,fHigh-resolution XPS spectra of Cu 2p(e) and Au 4f(f) for 7% Au–Cu/PTFE. The Gibbs free energy of adsorbed and non-adsorbed species ( G ) is calculated as 
    G=E+ZPE+ CpdT-TS
 (4) where E , ZPE, C p , and S are the electronic energy directly obtained from DFT calculations, zero-point energy, heat capacity, and entropy, respectively (see Supplementary Table 2 for more details). T is set to room temperature (298.15 K) for a better comparison with the experimental measurements. Electrode preparation All chemicals were used as received without further purification. All aqueous solutions were prepared using deionized water with a resistivity of 18.2 MΩ cm. The Cu/PTFE cathodes were prepared by sputtering 100 nm thickness of Cu catalysts (Cu target, 99.999%, Kurt J. Lesker company) on PTFE membranes (pore size: 450 nm, Beijing Zhongxingweiye Instrument Co., Ltd.) using a magnetron sputtering system. In the cathode, a porous PTFE membrane functions as a stable hydrophobic gas diffusion layer and prevents flooding during operation [7] . 3% Au–Cu, 7% Au–Cu, and 10% Au–Cu cathodes were prepared by immersing the Cu/PTFE electrodes in N 2 -saturated HAuCl 4 aqueous solution (5 μmol L −1 ) at 40 °C for 30 min, 65 °C for 15 min, and 65 °C for 30 min, respectively. Ag/AgCl reference electrode (3 M KCl, BASi) and Ni foam (1.6 mm thickness, MTI Corporation) was used as the reference electrode and anode, respectively. Ni foam was used as an OER electrode in the anode due to its commercial availability and good stability [35] , [63] . Material characterization. SEM images and the corresponding EDX elemental mapping were taken using the Hitachi FE-SEM SU5000 microscope. HAADF-STEM and bright-field STEM images, and the corresponding EDX elemental mapping were taken using a Hitachi HF-3300 microscope at 300 kV. XRD was recorded on Rigaku SmartLab X-ray diffractometer with Cu-K α radiation. The surface compositions of electrodes were determined by XPS (Thermo Scientific K-Alpha) using a monochromatic aluminum X-ray source. Operando Cu K-edge XAS spectra recorded in fluorescence yield were performed at the SuperXAS beamline at the Swiss Light Source. Ex situ XAS measurements were carried out at the Advanced Photon Source (Argonne National Laboratory). XAS data were processed by Athena and Artemis software included in a standard IFEFFIT package [64] . Electrochemical measurements The electrochemical measurements were conducted in an electrochemical flow cell setup configuration with the three-electrode system at an electrochemical station (AUT50783). The geometric area of the cathode in the flow cell is 1 cm 2 , which is used for all current density calculations. 30 mL of CO 2 -saturated 1 M KHCO 3 aqueous solution was introduced into the cathode chamber and the anode chamber at the rate of 10 mL min −1 by two pumps, respectively. An anion exchange membrane (Fumasep FAB-PK-130, Fuel Cell Store) was used to separate the cathode chamber and anode chamber. Pure CO 2 gas (Linde, 99.99%) or N 2 -diluted CO 2 gas with different CO 2 concentrations (75% and 84%) was continuously supplied to the gas chamber of the flow cell at a flow rate of 90 mL min −1 . The CO 2 RR performance was tested using constant-current electrolysis while purging CO 2 into the catholyte during the whole electrochemical test. The potentials vs. Ag/AgCl reference electrode were converted to values vs. reversible hydrogen electrode using the equation 
    E_RHE=E_Ag/AgCl+0.210 V+0.0591×pH
 (5) The ohmic loss between the working and reference electrodes was evaluated by electrochemical impedance spectroscopy technique and 80% i R compensation was applied to correct the potentials manually. Gas products were analyzed using a gas chromatograph (PerkinElmer Clarus 600) equipped with thermal conductivity and flame ionization detectors. Liquid products were analyzed by nuclear magnetic resonance spectrometer (Agilent DD2 600 MHz) and dimethylsulfoxide was used as an internal standard. We calculated the methane cathodic EE based on the equation as follows [7] : 
    Cathodic EE=(1.23+(-E_methane))× FE_methane/(1.23+(-E_applied)),
 (6) where the overpotential of oxygen evolution is assumed to be 0, E applied is the potential used in the experiment, FE methane is the measured Faradaic efficiency of methane in percentage, and E methane = 0.17 V RHE for CO 2 RR (ref. [65] ).